Taming the stability of Pd active phases through a compartmentalizing strategy toward nanostructured catalyst supports The design and synthesis of robust sintering-resistant nanocatalysts for high-temperature oxidation reactions is ubiquitous in many industrial catalytic processes and still a big challenge in implementing nanostructured metal catalyst systems. Herein, we demonstrate a strategy for designing robust nanocatalysts through a sintering-resistant support via compartmentalization. Ultrafine palladium active phases can be highly dispersed and thermally stabilized by nanosheet-assembled γ-Al 2 O 3 (NA-Al 2 O 3 ) architectures. The NA-Al 2 O 3 architectures with unique flowerlike morphologies not only efficiently suppress the lamellar aggregation and irreversible phase transformation of γ-Al 2 O 3 nanosheets at elevated temperatures to avoid the sintering and encapsulation of metal phases, but also exhibit significant structural advantages for heterogeneous reactions, such as fast mass transport and easy access to active sites. This is a facile stabilization strategy that can be further extended to improve the thermal stability of other Al 2 O 3 -supported nanocatalysts for industrial catalytic applications, in particular for those involving high-temperature reactions. The development of thermally robust supported metal nanocatalysts that can undergo high-temperature oxidative or reductive processes is of great interest for industrial catalytic reactions, such as catalytic combustion of hydrocarbons at elevated temperatures and water-gas shift reactions under high temperatures and pressures [1] , [2] , [3] , [4] , [5] , [6] , [7] , [8] , [9] , [10] , [11] , [12] . However, owing to their low Tammann temperatures and high surface energies, catalytically active metal nanoparticles are thermodynamically unstable and tend to sinter or coalescence into larger particles during reactions, especially at high reaction temperatures [13] , [14] , [15] , [16] . In addition, phase transformations or the structural collapse of supports at elevated temperatures may exacerbate the sintering or encapsulation of metal nanoparticles [17] , [18] , [19] . Unfortunately, both such thermal behaviours will result in fast deactivation of the catalysts and thus hamper their practical applications in industry. To obtain a sintering-resistant supported nanocatalyst, it is essential to address these issues by employing a suitable host support that can strengthens the metal-support interaction to stabilize metal nanoparticles and provides good mechanical stability to maintain the structural integrity at elevated temperatures [20] , [21] , [22] , [23] , [24] , [25] , [26] , [27] , [28] , [29] , [30] . Gamma phase alumina (γ-Al 2 O 3 ) is one of the most popular industrial catalysts and catalyst supports because of its compact crystal structure, excellent mechanical strength, high thermal stability, and robust chemical inertness [31] , [32] , [33] . Recently, it has been proved by high-resolution 27 Al nuclear magnetic resonance ( 27 Al NMR) that the coordinatively unsaturated pentacoordinate Al 3+ (Al 3+ penta ) centers present in γ-Al 2 O 3 can act as binding sites for anchoring metals [34] . This finding is important in which it provides a facile approach to preparing thermally robust supported metal nanocatalysts [35] , [36] . To better utilize these Al 3+ penta centers to stabilize metals, two-dimensional (2D) γ-Al 2 O 3 nanosheets with open surface structures were synthesized [37] , [38] , [39] . However, because of their huge surface energies, these free-standing γ-Al 2 O 3 nanosheets (N-Al 2 O 3 ) tended to stack or agglomerate as bulk ones at elevated temperatures, or even under reaction [40] . This behavior not only induced the loss of the unique structural benefits of nanosheets for heterogeneous catalysis but also, more seriously, resulted in the sintering and/or encapsulation of metal nanoparticles, which rapidly deactivated the catalysts (Fig. 1 ). Therefore, finding a way to prevent the lamellar aggregation of nanosheets to preserve their unique electronic and structural advantages for stabilizing metals is of significant importance for the fabrication of thermally stable γ-Al 2 O 3 nanosheet-supported catalysts. Fig. 1 Illustration of stabilization of Pd active phases . a Pd active phases stabilized by N-Al 2 O 3 in air at 1000 °C. b Pd active phases stabilized by NA-Al 2 O 3 in air at 1000 °C Full size image The hierarchical assembly of 2D nanosheets into three-dimensional (3D) configurations can efficiently overcome the huge surface energies to prevent lamellar stacking, which is clearly demonstrated by the development of 3D graphene, flowerlike TiO 2 flakes and nanospherical carbon nitride nanosheet frameworks, and other structures [41] , [42] , [43] , [44] , [45] , [46] , [47] , [48] . Inspired by this kind of structural arrangement, γ-Al 2 O 3 nanosheets dominated by (110) facets are cross-linked as a hierarchical architecture with a unique flowerlike morphology (Fig. 1 ). For nanosheet-assembled Al 2 O 3 (NA-Al 2 O 3 ), the interconnected topology of the nanosheets provides enough structural rigidity against the surface energies to perfectly stabilize γ-Al 2 O 3 nanosheets against lamellar aggregation and maintain the (110) facets at elevated temperatures. In addition, the thermally induced irreversible γ-to-α phase transformation is efficiently inhibited by spatially separating the nanosheets from each other to block the surface-controlled phase reactions (Supplementary Fig. 1 ). As a result, the NA-Al 2 O 3 architecture serves as a robust host material with unique structural benefits to support metal nanoparticles, and the resultant nanocatalyst exhibits excellent thermal stability and hierarchical structural benefits for heterogeneous catalysis. For example, the Al 3+ penta centers can serve as anchor sites to immobilize ultrafine metal nanoparticles on nanosheets with a strong metal-support interaction [34] , [35] , [36] . And the robust structural interconnectivities of the 3D architecture afford enough mechanical stability to protect the structural integrity against deformation and phase transformation at elevated temperatures, thus efficiently avoiding the sintering and encapsulation of metal nanoparticles caused by support material deformation [49] , [50] , [51] , [52] . Furthermore, the flowerlike morphology, with its multifaceted open surfaces, is favorable for mass transfer and made the active metal phases more easily accessible to the reacting molecules. Experimentally, both characteristics are beneficial for heterogeneous catalysis. Hence, it is significant that the ultrafine metals supported on the NA-Al 2 O 3 architecture are thermally robust for high-temperature oxidative or reductive reactions. Herein, NA-Al 2 O 3 hierarchical architectures are fabricated and employed as the host materials to disperse and stabilize ultrafine palladium (Pd) active phases (Pd/NA-Al 2 O 3 ) for high-temperature oxidative reactions. As a result of its robust thermal stability, Pd/NA-Al 2 O 3 exhibits an excellent catalytic performance toward combustion of hydrocarbons (e.g. methane and propane) at elevated temperatures. Furthermore, this facile stabilization strategy can be further extended to improve the thermal stability of other Al 2 O 3 -supported nanocatalysts for industrial catalytic applications, in particular for those involving high-temperature reactions. Thermal behavior of NA-Al 2 O 3 architectures Fig. 2 illustrates the thermal stability of NA-Al 2 O 3 . To evaluate the thermal behavior, the as-prepared NA-Al 2 O 3 architectures were subjected to an annealing treatment at 1000 °C in air for 3 h (the resultant sample was denoted as NA-Al 2 O 3 -1000) and then were characterized by means of scanning electron microscopy (SEM), transmission electron microscopy (TEM), atomic force microscope (AFM), N 2 -sorption analysis, and X-ray diffraction (XRD). In Fig. 2a and Supplementary Fig. 2 , the as-prepared NA-Al 2 O 3 architectures were assembled from ~5-nm-thick flat nanosheets in a highly interconnected fashion to form a hollow spherical morphology; their diameters and shell thicknesses were determined to be 3–6 μm and 500–900 nm, respectively. Benefiting from the structural and mechanical advantages of such cross-linked nanosheet networks, which protected against lamellar aggregation, the hierarchical hollow architecture of NA-Al 2 O 3 was quite robust and sustained 1000 °C annealing in air for 3 h without deformation (Fig. 2b and Supplementary Fig. 3 ). The specific surface area (S BET ) of NA-Al 2 O 3 and NA-Al 2 O 3 -1000 was determined to be 219 and 148 m 2 g −1 (Supplementary Fig. 4 ), indicating that NA-Al 2 O 3 has an excellent thermal stability comparable to commercial La-doped γ-Al 2 O 3 (La-Al 2 O 3 , S BET = 152 m 2 g −1 for La-Al 2 O 3 , S BET = 107 m 2 g −1 for La-Al 2 O 3 -1000, Supplementary Fig. 5 ). In addition, the surface structure of the NA-Al 2 O 3 also became much more open after the 1000 °C-annealing, which should be kinetically favorable for heterogeneous reactions. On the contrary, obvious structural deformation, particularly layer restacking/agglomeration occurred in the free-standing N-Al 2 O 3 (Supplementary Fig. 6 ). It resulted in the evident decrease of S BET from 198 to 78 m 2 g −1 , seriously counteracting the structural advantages of the nanosheet morphology for heterogeneous catalysis. The crystallinity of NA-Al 2 O 3 was greatly improved by 1000 °C-annealing treatment, as indicated by the appearance of high-resolution XRD reflections at 32.8, 37.1, and 39.5, respectively, for (220), (311), and (222) γ-Al 2 O 3 (Fig. 2c , JCPDS 10-0425). As a result of the spatial separation of the nanosheets from each other to block the surface-controlled phase reactions, the thermally induced phase transformation was well suppressed on the NA-Al 2 O 3 architecture; whereas for N-Al 2 O 3 , an irreversible γ-to-θ phase transformation was observed after calcination in air at 1000 °C for 3 h (Fig. 2c vs. Supplementary Fig. 7 ). To further investigate the thermal stability of NA-Al 2 O 3 , its hierarchical architectures were deformed by mechanical grinding (denoted as NA-Al 2 O 3 -deformed) and then subjected to 1000 °C-annealing. Similar to the results obtained from N-Al 2 O 3 -1000, irreversible γ-to-θ phase transformation and significant decrease of S BET were observed for NA-Al 2 O 3 -deformed-1000 (S BET = 195 m 2 g −1 for NA-Al 2 O 3 -deformed, S BET = 72 m 2 g −1 for NA-Al 2 O 3 -deformed-1000, Supplementary Fig. 8 ), further demonstrating the important role of compartmentalization strategy in stabilizing 2D nanosheets from sintering and collapse. In Fig. 2d , the nanosheet was aligned to edge-on conditions, e.g. [112] zone axis of γ- Al 2 O 3 to study the terminal surfaces of NA-Al 2 O 3 [53] , [54] . As indicated by the clearly resolved lattice fringes of (2 \(\overline 2\) 0) and (11 \(\overline 1\) ) planes, the preferred surfaces of NA-Al 2 O 3 were (110) facets. A schematic diagram was also given to show the geometry of the nanosheet structure. Thus, we conclude that the NA-Al 2 O 3 architecture with primarily exposed (110) facets is a thermally robust host material and can be used to prepare sintering-resistant supported nanocatalysts. Fig. 2 Thermal characterization of NA-Al 2 O 3 host materials. a SEM images of NA-Al 2 O 3 . b SEM images of NA-Al 2 O 3 -1000. c XRD patterns of NA-Al 2 O 3 and NA-Al 2 O 3 -1000. d HRTEM image of a typical nanosheet of NA-Al 2 O 3 -1000. Upper panel: It was aligned to an edge-on condition, namely, a condition that the basal surfaces (2 \(\overline 2\) 0) of nanosheets were in parallel with the electron beam. The inset is the FFT pattern recorded from the nanosheet. Lower panel: A schematic diagram showing the geometry of the nanosheets. The two basal planes of the nanosheet are colored blue. The scale bar in ( a and b corresponds to 2 µm, and in d corresponds to 5 nm Full size image Thermal behavior of Pd/NA-Al 2 O 3 nanocatalysts The as-prepared NA-Al 2 O 3 architectures were directly used to support Pd active phases through an incipient wet impregnation method to load Pd species. To better demonstrate the outstanding ability of NA-Al 2 O 3 to stabilize metals, the metal loading was increased to 5 wt%, and the resultant sample was then subjected to annealing at 1000 °C in air for 3 h (the samples before and after 1000 °C-annealing are denoted Pd/NA-Al 2 O 3 and Pd/NA-Al 2 O 3 -1000, respectively). Owing to the excellent stability of the NA-Al 2 O 3 architecture (Fig. 2 ), Pd/NA-Al 2 O 3 nanocatalysts were sufficiently robust to maintain their structural integrity under 1000 °C-annealing, thus efficiently avoiding the sintering and encapsulation of Pd nanoparticles caused by nanostructural deformation (Fig. 3a vs. 3b ). The S BET of Pd/NA-Al 2 O 3 and Pd/NA-Al 2 O 3 -1000 was determined to be 152 and 145 m 2 g −1 , respectively (Supplementary Fig. 9 ). Such flowerlike hierarchical structure with well-preserved surface area was beneficial for Pd-catalyzed reactions because it facilitated the transport of reacting molecules to the surface of the catalyst to participate in the reaction [55] , [56] . The particle sizes of the Pd active phase were determined to be 2.6 ± 0.2 nm and 2.8 ± 0.2 nm for Pd/NA-Al 2 O 3 and Pd/NA-Al 2 O 3 -1000, respectively (Fig. 3c, d and Supplementary Fig. 9 ). This result clearly confirms that the Pd active phase can be well stabilized by NA-Al 2 O 3 against sintering at elevated temperatures. In sharp contrast, serious sintering of the Pd active phase with increasing the particle size from 2.5 ± 0.3 nm to 75.9 ± 17.7 nm and collapse of the Al 2 O 3 nanosheets with decreasing the S BET from 139 to 70 m 2 g −1 occurred in Pd/N-Al 2 O 3 , owing to the poor thermal stability of the free-standing nanosheet structure (Supplementary Fig. 10 ). In addition, NA-Al 2 O 3 with deformed nanostructure (Supplementary Fig. 8 ) was also used to support Pd species. In Supplementary Fig. 11 , evident sintering of Pd active phases also happened to Pd/NA-Al 2 O 3 -deformed-1000, further demonstrating that the compartmentalization of nanosheets plays a critical role in stabilizing Pd active phases. To better study the influence of phase change of alumina on stabilizing Pd species, La-Al 2 O 3 with an excellent thermal stability (Supplementary Fig. 5 ) was also employed for Pd loading. Similar to the results obtained from Pd/N-Al 2 O 3 -1000 and Pd/NA-Al 2 O 3 -deformed-1000, an obvious sintering behavior still happened to Pd/La-Al 2 O 3 -1000 (Supplementary Fig. 12 ). These three control experiments underline the structural advantages of nanosheet-assembly hierarchical architectures in stabilizing metals under elevated temperatures. In Supplementary Fig. 13 , Pd/NA-Al 2 O 3 , Pd/N-Al 2 O 3 , and Pd/La-Al 2 O 3 nanocatalysts were also subjected to an annealing treatment in wet air condition (10 vol% H 2 O) to evaluate their hydrothermal stability for practical catalytic applications. As expected, the ultrafine Pd active phases can be well still stabilized by NA-Al 2 O 3 even after calcinated in wet air, whereas significant sintering of Pd phases occurred to N-Al 2 O 3 and La-Al 2 O 3 supported samples. This finding demonstrated that Pd/NA-Al 2 O 3 is a promising nanocatalyst that can work under wet air conditions. Fig. 3 Thermal characterization of Pd/NA-Al 2 O 3 nanocatalysts. a SEM images of Pd/NA-Al 2 O 3 . b SEM images of Pd/NA-Al 2 O 3 -1000. c TEM images of Pd/NA-Al 2 O 3 . d TEM images of Pd/NA-Al 2 O 3 -1000. e XRD patterns of Pd/NA-Al 2 O 3 -1000 and Pd/NA-Al 2 O 3 . f Raman spectra of Pd/NA-Al 2 O 3 -1000 and Pd/NA-Al 2 O 3 . The scale bar in a and b corresponds to 2 µm, and in c and d corresponds to 50 nm Full size image Figure 3e shows the crystal structure of Pd/NA-Al 2 O 3 before and after thermal annealing. Using the unique structural benefits of the hierarchical architecture to suppress the thermally induced phase conversion confirmed that the γ phase was the predominant phase for the host NA-Al 2 O 3 in both samples. 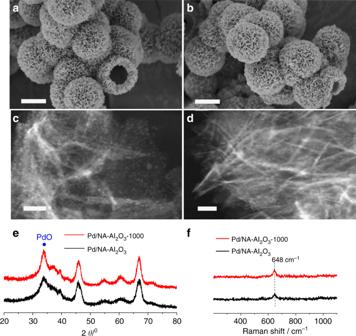Fig. 3 Thermal characterization of Pd/NA-Al2O3nanocatalysts.aSEM images of Pd/NA-Al2O3.bSEM images of Pd/NA-Al2O3-1000.cTEM images of Pd/NA-Al2O3.dTEM images of Pd/NA-Al2O3-1000.eXRD patterns of Pd/NA-Al2O3-1000 and Pd/NA-Al2O3.fRaman spectra of Pd/NA-Al2O3-1000 and Pd/NA-Al2O3. The scale bar inaandbcorresponds to 2 µm, and incanddcorresponds to 50 nm The new diffraction peaks arising at 33.8 and 54.7° were identified as the characteristic (101) and (112) reflections of palladium oxide (PdO), and no other peak assigned to metallic Pd was observed [57] , [58] . This finding indicates that the Pd active phase was stabilized mainly as PdO nanoparticles on NA-Al 2 O 3 , even after harsh high-temperature treatment, rather than Pd nanoparticles. 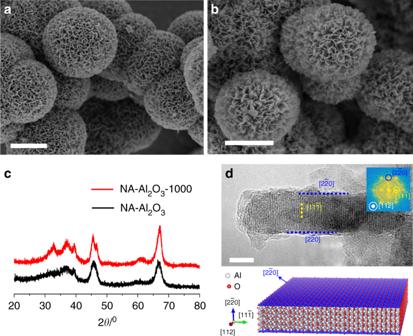It was further confirmed by Raman spectra. Fig. 2 Thermal characterization of NA-Al2O3host materials.aSEM images of NA-Al2O3.bSEM images of NA-Al2O3-1000.cXRD patterns of NA-Al2O3and NA-Al2O3-1000.dHRTEM image of a typical nanosheet of NA-Al2O3-1000. Upper panel: It was aligned to an edge-on condition, namely, a condition that the basal surfaces (2\(\overline 2\)0) of nanosheets were in parallel with the electron beam. The inset is the FFT pattern recorded from the nanosheet. Lower panel: A schematic diagram showing the geometry of the nanosheets. The two basal planes of the nanosheet are colored blue. The scale bar in (aandbcorresponds to 2 µm, and indcorresponds to 5 nm In Fig. 3f , the formation of PdO on NA-Al 2 O 3 is clearly identified by the appearance of a characteristic peak assigned to the B 1g mode of Pd-O at a Raman shift of 648 cm −1 [59] , [60] . This finding is apparently inconsistent with the fact that PdO will transform into metallic Pd when being subjected to 1000 °C-annealing in air [61] , [62] . To better solve this issue, a control experiment that cooling down the Pd/NA-Al 2 O 3 nanocatalyst in N 2 was carried out after annealing the sample at 1000 °C in air. As demonstrated in Supplementary Fig. 14 , the high-temperature induced decomposition of PdO indeed happened to Pd/NA-Al 2 O 3 nanocatalyst, and the PdO was partially transformed into metallic Pd when cooled down in N 2 . But why is only PdO phase determined in Pd/NA-Al 2 O 3 -1000? The reason should be mainly attributed to that Pd active phases can be well stabilized in ultrasmall size by NA-Al 2 O 3 (Supplementary Fig. 9 ), which facilitates the completely reoxidization of metallic Pd back to PdO phase by air during the cooling process. This finding was further confirmed by the results obtained from N-Al 2 O 3 , La-Al 2 O 3 , and NA-Al 2 O 3 -deformed supported samples. 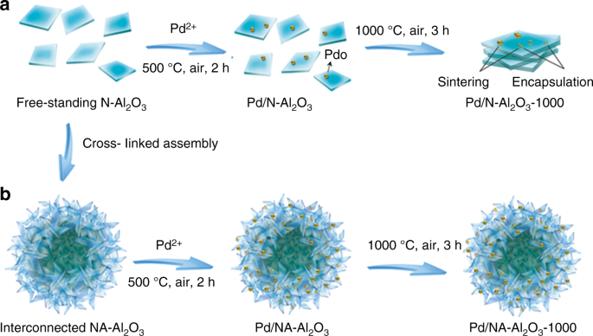In Supplementary Fig. 15 , owing to the evident sintering of Pd active phases, the arising of metallic Pd reflection at 40.1° was observed on Pd/N-Al 2 O 3 -1000, Pd/La-Al 2 O 3 -1000 and Pd/NA-Al 2 O 3 -deformed-1000 samples, indicating that PdO had been partially transformed into metallic Pd, even when they were cooled down in air. Fig. 1 Illustration of stabilization of Pd active phases. aPd active phases stabilized by N-Al2O3in air at 1000 °C.bPd active phases stabilized by NA-Al2O3in air at 1000 °C The Pd dispersion of Pd/NA-Al 2 O 3 , Pd/N-Al 2 O 3 and Pd/La-Al 2 O 3 before and after the 1000 °C-annealing treatment was summarized in Supplementary Table 1 . Hence, it is clear that the Pd active phase was highly dispersed and stabilized as ultrasmall PdO nanoparticles by NA-Al 2 O 3 at elevated temperatures in air, so supported Pd species in the oxidation state were favorable for high-temperature oxidation reactions. It should be noted that if PdO active phases had been previously reduced by H 2 , the resultant metallic Pd nanoparticles can be also well stabilized by NA-Al 2 O 3 from sintering, even after 1000 °C-annealing in N 2 (Supplementary Fig. 16a ). In sharp comparison, sintering of metallic Pd was observed on N-Al 2 O 3 and La-Al 2 O 3 supported nanocatalysts (Supplementary Fig. 16b, c ). Hence, by taking advantage of the unique nanostructure of NA-Al 2 O 3 , in particular compartmentalized 2D nanosheets with enlarged surface structure, Pd active species, either in oxidative or metallic phases can be well stabilized by NA-Al 2 O 3 at elevated temperatures. Strong interaction between PdO and NA-Al 2 O 3 In Fig. 4 , the interaction between PdO and NA-Al 2 O 3 is investigated by 2D 27 Al NMR spectra, high-resolution (HR)-TEM imaging, and theoretical calculation. In the NMR spectra, three distinct peaks centered at 7, 32, and 65 ppm chemical shifts are observed on the as-prepared NA-Al 2 O 3 host materials (Fig. 4a ), which were assigned to the Al 3+ ions in octahedral (Al 3+ octa ), pentahedral (Al 3+ penta ) and tetrahedral (Al 3+ tetra ) coordination, respectively [63] , [64] , [65] . Among them, the Al 3+ penta sites are considered as the primary anchoring sites for active catalytic phases and should play an essential role in the dispersion and stabilization of Pd oxide species [34] , [35] , [36] . Upon loading of the PdO on NA-Al 2 O 3 , the intensity of the peak Al 3+ penta decreased significantly, indicating that most of the Al 3+ penta sites had been used to immobilize Pd oxides on Al 2 O 3 nanosheets (Fig. 4b ) [37] . In Fig. 4c , the growth of PdO onto Al 2 O 3 is confirmed by the HRTEM images, where Pd active phases sitting on the (110) surfaces of γ-Al 2 O 3 nanosheets was clearly resolved. The energetics of the interaction of PdO with the (110) facets of γ-Al 2 O 3 were studied by theoretical calculations In Fig. 4d , the sitting of PdO on (110) facets of γ-Al 2 O 3 is exothermic, and the corresponding adsorption energy is determined to be 3.16 eV. This finding suggested that the Pd active phase supported on the (110) facets of γ-Al 2 O 3 is thermodynamically stable, and large energy would be required for Pd-O bond breaking if the Pd phase started to migrate and sinter. Hence, the (110) facets of γ-Al 2 O 3 thermodynamically facilitated the stabilization of the Pd active phase against sintering. The preservation of the structural integrity of γ-Al 2 O 3 nanosheets to retain their (110) facets is therefore favorable for the preparation of robust sintering-resistant catalysts. Fig. 4 Structural characterization of NA-Al 2 O 3 and Pd/NA-Al 2 O 3 . a Two-dimensional 27 Al MQ MAS NMR spectra of NA-Al 2 O 3 . b Two-dimensional 27 Al MQ MAS NMR spectra of Pd/NA-Al 2 O 3 . c TEM image of Pd/NA-Al 2 O 3 -1000. d Calculated structure of Pd/NA-Al 2 O 3 . The scale bar in c corresponds to 5 nm Full size image Catalytic performance in methane combustion Owing to the unique catalytic ability of Pd species in oxidation reactions, synthesized Pd/Al 2 O 3 catalysts were subjected to methane oxidation at elevated temperatures for the purpose of better evaluating their catalytic performance, particularly thermal stability and catalytic durability. In Fig. 5a , obvious size-dependent catalytic behavior toward methane oxidation was observed on Pd/Al 2 O 3 nanocatalysts. For example, a significant loss of activity was determined for Pd/N-Al 2 O 3 and Pd/La-Al 2 O 3 after 1000 °C-annealing, which was due to the evident growth and/or encapsulation of PdO under high temperatures (Pd/N-Al 2 O 3 vs. Pd/N-Al 2 O 3 -1000, and Pd/La-Al 2 O 3 vs. Pd/La-Al 2 O 3 -1000). In contrast, the catalytic activity of Pd/NA-Al 2 O 3 was actually slightly better after thermal annealing (Pd/NA-Al 2 O 3 vs. Pd/NA-Al 2 O 3 -1000). According to the literature, this improved performance is attributable to the good stabilization of PdO nanoparticles without sintering and the strengthening of the metal-support interaction by high-temperature annealing [66] , [67] , [68] , [69] . In Supplementary Fig. 17, a similar size-dependent catalytic behavior toward propane combustion was also observed, further confirming the thermal-induced size evolution of PdO nanoparticles in these nanocatalysts. To evaluate their catalytic stability, several control experiments were carried out. First are the successive ignition-extinction cycles for methane oxidation. For Pd/NA-Al 2 O 3 , the catalytic performance was rather robust without activity loss over five runs (Fig. 5b ); whereas for Pd/N-Al 2 O 3 and Pd/La-Al 2 O 3 , a significant loss of activity toward to a higher reaction temperature occurred immediately in the second run (Supplementary Fig. 18 ), due to the sintering of PdO nanoparticles at the first run. To indicate the stability under hydrothermal condition, water vapor (~10 vol%) was introduced to the reaction system. In Supplementary Fig. 19 , Pd/NA-Al 2 O 3 still exhibited a robust catalytic durability over Pd/N-Al 2 O 3 and Pd/La-Al 2 O 3 nanocatalysts for the catalytic combustion of methane in the present of water (~10 vol%), because of its sintering-resistant PdO nanoparticles in wet air (Supplementary Fig. 13 ). To demonstrate that PdO phases are stabilized during methane combustion, the heating/cooling ramps were collected. In Fig. 5c and Supplementary Fig. 20 , the typical hysteresis curve caused by PdO-Pd-PdO transformation during cooling process was absent in all Pd/Al 2 O 3 nanocatalysts, indicating that Pd active phases had been well stabilized in oxidative state for methane oxidation [70] . As a result of being heated to a higher temperature (850 vs. 450 °C) to induce obvious sintering, the activity loss of Pd/N-Al 2 O 3 and Pd/La-Al 2 O 3 became much more evidence in the light-off curves (Fig. 5a vs Supplementary Fig. 20 ). To better study the influence of reaction temperatures on catalytic activity, long-term operation of methane combustion at alternating reaction temperatures (e.g. 300-800-300 °C) was carried out. In Fig. 5d , each of the three catalysts exhibited a comparable catalytic stability in the first 10 h-run at 300 °C; but after being accelerated aging at 800 °C for 5 h, a significant loss of activity was observed for Pd/N-Al 2 O 3 and Pd/La-Al 2 O 3 when ramping the reaction temperature back to 300 °C. Interesting, Pd/NA-Al 2 O 3 demonstrated a robust catalytic durability during this process. Hence, it can be concluded that the nanosheet-interconnected hierarchical architecture played an essential role in stabilizing PdO nanoparticles for catalysis, and the resultant Pd/NA-Al 2 O 3 was a robust sintering-resistant catalyst suitable for high-temperature oxidation reactions (Supplementary Fig. 21 ). Fig. 5 Catalytic combustion of methane on Pd/Al 2 O 3 nanocatalysts. a CH 4 conversion vs reactor temperature. b Repeating ignition−extinction cycles of methane conversion on Pd/NA-Al 2 O 3 . c Light-off curves of methane conversion on Pd/NA-Al 2 O 3 at temperatures between 100–850 °C. 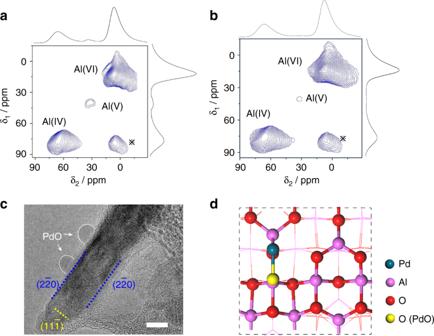Fig. 4 Structural characterization of NA-Al2O3and Pd/NA-Al2O3.aTwo-dimensional27Al MQ MAS NMR spectra of NA-Al2O3.bTwo-dimensional27Al MQ MAS NMR spectra of Pd/NA-Al2O3.cTEM image of Pd/NA-Al2O3-1000.dCalculated structure of Pd/NA-Al2O3. The scale bar inccorresponds to 5 nm 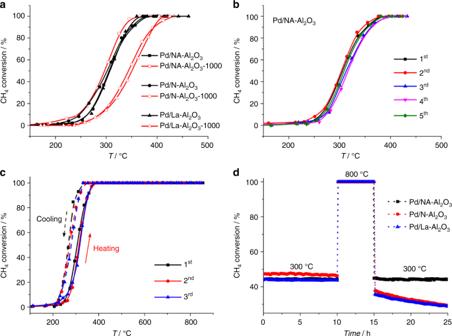Fig. 5 Catalytic combustion of methane on Pd/Al2O3nanocatalysts.aCH4conversion vs reactor temperature.bRepeating ignition−extinction cycles of methane conversion on Pd/NA-Al2O3.cLight-off curves of methane conversion on Pd/NA-Al2O3at temperatures between 100–850 °C.dLong-term combustion of methane at 300-800-300 °C on Pd/NA-Al2O3, Pd/N-Al2O3and Pd/La-Al2O3 d Long-term combustion of methane at 300-800-300 °C on Pd/NA-Al 2 O 3 , Pd/N-Al 2 O 3 and Pd/La-Al 2 O 3 Full size image In this study, we demonstrated that ultrafine Pd active phases were well stabilized by an NA-Al 2 O 3 architecture as a promising sintering-resistant nanocatalyst for high-temperature oxidation reactions. Such cross-linked γ-Al 2 O 3 nanosheets with flowerlike morphologies provided enough structural rigidity to efficiently suppress lamellar aggregation and the irreversible phase transformation of γ-Al 2 O 3 nanosheets at elevated temperatures to avoid the sintering and encapsulation of Pd active phases. In addition, the flowerlike morphologies with multifaceted open surfaces demonstrated significant structural advantages for heterogeneous reactions, such as fast mass transport and easily accessible active sits. As a result, Pd/NA-Al 2 O 3 nanocatalysts exhibited excellent catalytic activity and durability for methane combustion at high temperatures. We hope this facile synthetic strategy can be further extended to improve the thermal stability of other Al 2 O 3 -supported nanocatalysts for industrial catalytic applications, particularly those involving high-temperature reactions. Synthesis of nanosheet-assembled Al 2 O 3 (NA-Al 2 O 3 ) In all, 1.51 g of Al(NO 3 ) 3 ·9H 2 O, 0.70 g of K 2 SO 4 , and 0.50 g of CO(NH 2 ) 2 were dissolved in 80 mL deionized water. Then the obtained mixture was transferred into a 100 mL Teflon-lined stainless steel autoclave and heated at 180 °C for 3 h. When cooled to room temperature, the white precipitate was collected by filtration, dried at 80 °C for 12 h and finally calcined at 500 °C for 2 h. Synthesis of Al 2 O 3 nanosheet (N-Al 2 O 3 ) The typical procedure to synthesize thin alumina nanosheet was as follows: 0.60 g of Al(NO 3 ) 3 ·9H 2 O, 0.24 g of lysine, and 0.77 g of CO(NH 2 ) 2 were dissolved in 80 mL deionized water to form a homogeneous solution under magnetic stirring. Then the solution was transferred into a 100 mL Teflon-lined stainless autoclave and heated at 100 °C for 24 h. After cooled to room temperature, the white precipitate was filtered, washed with deionized water and anhydrous alcohol several times, and then dried at 80 °C for 12 h. The sample was gained after calcination of the powder in air at 500 °C for 2 h with a heating rate of 1 °C min −1 . Preparation of Pd/NA-Al 2 O 3 5 wt% Pd active phases were loaded on NA-Al 2 O 3 by incipient wet impregnation method and dried at 80 °C for 12 h. The obtained samples were then calcined at 500 °C for 2 h. Pd/N-Al 2 O 3 and Pd/La-Al 2 O 3 were prepared with the same method. Preparation of Pd/NA-Al 2 O 3 -1000 The as-prepared Pd/NA-Al 2 O 3 , Pd/N-Al 2 O 3 , and Pd/La-Al 2 O 3 were calcined at 1000 °C for 3 h. Pd/N-Al 2 O 3 -1000 and Pd/La-Al 2 O 3 -1000 were prepared with the same method. Characterization The powder X-ray diffraction (XRD) patterns were collected on a Bruker D8 Focus diffractometer with Cu Kα radiation ( λ = 1.54056 Ǻ, operated at 40 kV and 40 mA). The X-ray photoelectron spectroscopy (XPS) were obtained at 25 °C on a PHI-Quantera SXM spectrometer with Al Kα (1486.6 eV) radiation as the excitation source at ultra-high vacuum (6.7 × 10 −8 Pa). All binding energies (BE) were determined with respect to the C1s line (284.8 eV) originating from adventitious carbon. The morphologies of samples were investigated by the field emission scanning electron microscopy (FE-SEM) images obtained by a NOVA NanoSEM 450 instrument operated at the beam energy of 5 kV. High-angle annular dark-field (HAADF) scanning transmission electron microscopy (STEM) images and high resolution TEM images were obtained on a JEM-ARM200F TEM/STEM with a guaranteed resolution of 0.08 nm. Before microscopy examination, the catalyst powders were ultrasonically dispersed in ethanol and then a drop of the solution was put onto a copper grid coated with a thin lacey carbon film. Raman spectra were recorded on a Renishaw Raman spectrometer under ambient conditions, and the 514 nm line of a Spectra Physics Ar + laser was used for an excitation. The laser beam intensity was 2 mW, and the spectrum slit width was 3.5 cm −1 . Solid state 27 Al MAS NMR was performed at room temperature on a Bruker AVANCE III 500 MHz solid-state NMR spectrometer, operating at a magnetic field of 11.7 T. The corresponding 27 Al Larmor frequency was 130.28 MHz. All spectra were recorded at a sample spinning rate of 4 kHz. Each spectrum was acquired using a total of 2000 scans with a recycle delay time of 0.5 s and an acquisition time of 0.018 s. All spectra were externally referenced (i.e., the 0 ppm position) to an 1 M Al(NO 3 ) 3 aqueous solution. The Pd dispersion was measured by CO chemisorption method on the Autochem 2920 II apparatus. Before the test, the sample was pretreated in a flow (40 mL min −1 ) of 20 vol% O 2 balanced with Ar at 500 °C for 1 h. Then the sample was first reduced in a flow (40 mL min −1 ) of 5 vol% H 2 balanced with N 2 at 200 °C for 1 h. After cooled to room temperature in a flow of He (40 mL min −1 ), several pulses of CO (1 vol% CO balanced with He) were introduced into the sample until no more adsorption was observed. The stoichiometry for Pd: CO was taken be unity. Computational method and models Density functional theory (DFT) calculations were carried out using the Vienna Ab-initio Simulation Package (VASP). The spin-polarized projector augmented wave (PAW) method and the Perdew-Burke-Ernzerhof (PBE) electron exchange-correlation functional of the generalized gradient approximation (GGA) were applied in our calculations. The kinetic energy cut-off for the wave function expanded in the plane-wave basis was set as 400 eV. To optimize the structures, the calculation was performed until the maximum force upon each relaxed atom was less than 0.05 eV Å −1 . The vacuum height was set as 10 Å to eliminate the interaction between neighboring slabs. The adsorption energy ( E ads ) was calculated as followed Eq. ( 1 ): 
    E_ads =  - ( E_substrate + E_PdO - E_total)
 (1) where E total is the calculated total energy of the adsorption PdO cluster, E substrate is the energy of the clean substrate and E PdO is the energy of optimized PdO cluster in the vacuum. In order to study the adsorption of PdO cluster on γ-Al 2 O 3 (110) surfaces, we used the following model: a 1 × 2 surface cell was used to construct a four-atomic-layer Al 2 O 3 (110) slab, and the top three layers of the Al 2 O 3 (110) slab were allowed to relax. The Brillouin-zone integration was performed along with a 2 × 2 × 1 Monkhorst-Pack grid for the (110) surface slabs. Catalytic combustion of methane and propane The catalytic activity of the catalyst for CH 4 combustion was evaluated in a fixed-bed reactor containing 200 mg of catalyst at atmospheric pressure, and the feed gas consisted of 1 vol% CH 4 , 20 vol% O 2 , 10 vol% H 2 O (when used) and Ar. The total gas flow rate was 50 mL min −1 , and the corresponding gas hourly space velocity (GHSV) was 15 000 mL h −1 g cat −1 . The inlet and outlet CH 4 concentration were measured by Agilent GC 7890 A. The CH 4 conversion (X CH4 ) was calculated using the following Eq. ( 2 ): 
    X_CH_4% = [ CH_4]_in - [ CH_4]_out/[ CH_4]_in× 100
 (2) where [CH 4 ] in and [CH 4 ] out are the CH 4 concentrations in the inlet and outlet gas, respectively. The catalytic activity of the catalyst for C 3 H 8 combustion was evaluated in a fixed-bed reactor containing 100 mg of catalyst at atmospheric pressure, and the feed gas consisted of 0.2 vol% C 3 H 8 , 2 vol% O 2 , and Ar. The total gas flow rate was 50 mL/min, and the corresponding GHSV was 30 000 mL h −1 g cat −1 . The inlet and outlet C 3 H 8 concentration were measured by by an online gas chromatograph (GC-2060) that was equipped with an FID. The C 3 H 8 conversion (X C3H8 ) was calculated using the following Eq. ( 3 ): 
    X_C_3H_8% = [ C_3H_8]_in - [ C_3H_8]_out/[C_3H_8]_in× 100
 (3) where [C 3 H 8 ] in and [C 3 H 8 ] out are the C 3 H 8 concentrations in the inlet and outlet gas, respectively.